Stereoselective synthesis of sulfur-containing β-enaminonitrile derivatives through electrochemical Csp3–H bond oxidative functionalization of acetonitrile Incorporation of nitrile groups into fine chemicals is of particular interest through C(sp 3 )–H bonds activation of alkyl nitriles in the synthetic chemistry due to the highly efficient atom economy. However, the direct α-functionalization of alkyl nitriles is usually limited to its enolate chemistry. Here we report an electro-oxidative C(sp 3 )–H bond functionalization of acetonitrile with aromatic/aliphatic mercaptans for the synthesis of sulfur-containing β-enaminonitrile derivatives. These tetrasubstituted olefin products are stereoselectively synthesized and the stereoselectivity is enhanced in the presence of a phosphine oxide catalyst. With iodide as a redox catalyst, activation of C(sp 3 )–H bond to produce cyanomethyl radicals proceeds smoothly at a decreased anodic potential, and thus highly chemoselective formation of C–S bonds and enamines is achieved. Importantly, the process is carried out at ambient temperature and can be easily scaled up. Nitriles are widely found in pharmaceuticals, natural products, and materials [1] , [2] , [3] , [4] . Introduction of nitrile groups onto target frameworks by C–H functionalization of C(sp 3 )–H bonds of simple aliphatic nitriles is of particular interest in the synthetic chemistry. Early research has focused on the C–H activation of alkyl nitriles using stoichiometric amounts of transition metal salts (such as Ru, Rh, Ni, Fe, etc.) [5] , [6] , [7] , [8] , [9] . On the other hand, the direct α-functionalization of alkyl nitriles is usually limited to its enolate chemistry, which requires a strong base for its formation [10] , [11] , [12] , [13] , [14] , [15] . Recently, free radical-initiated α-C–H functionalization of alkyl nitriles has attracted attention (Fig. 1a ) [16] , [17] . Nevertheless, these methods require excess equivalents of strong oxidants (peroxides), metal-based oxidants (Ag + , Mn 3+ ), or single-electron transfer reagents (diazonium salts). In addition, all of these works were carried out at elevated temperatures. Therefore, methods for the mild and environmentally friendly activation of alkyl nitriles are still highly desirable. Fig. 1 Strategies for the formation of nitrile-containing alkyl radicals. a The formation of nitrile-containing alkyl radicals under traditional organic chemical or photochemical conditions. b The formation of cyanomethyl radicals under electrochemical conditions Full size image Electrochemical anodic oxidation represents an attractive and environment-friendly synthetic strategy to solve lingering problems in organic chemistry [18] , [19] , [20] , [21] , [22] , [23] , [24] , [25] , [26] , [27] , [28] , [29] , [30] , [31] , [32] , [33] . Particularly, the indirect electrolysis, in which a redox catalyst is utilized as the electron shuttle, achieves higher energy efficiency and different selectivity [34] , [35] , [36] , [37] , [38] , [39] , [40] , [41] , [42] , [43] . In continuation of our interest in the development of electrochemical methods to organic synthesis [44] , [45] , [46] , [47] , herein, we report the electrochemical C(sp 3 )–H bond oxidative functionalization of acetonitrile mediated by potassium iodide to synthesize sulfur-containing β-enaminonitrile derivatives highly efficiently in one pot (Fig. 1b ). Reaction optimization To initiate the investigation, p -fluorothiophenol ( 1aa ) and acetonitrile were chosen as the substrates to test the reaction. 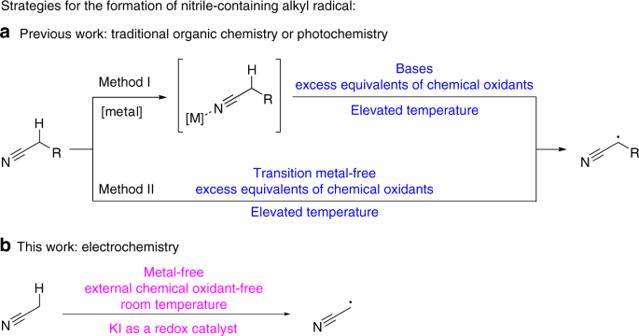Fig. 1 Strategies for the formation of nitrile-containing alkyl radicals.aThe formation of nitrile-containing alkyl radicals under traditional organic chemical or photochemical conditions.bThe formation of cyanomethyl radicals under electrochemical conditions Under a galvanostatic condition at 10 mA in an undivided cell, the reaction of 1aa and acetonitrile with 10 mol% citric acid, 20 mol% 1,2-bis(diphenylphosphino)ethane (DPPE), and 50 mol% KI gave a 96% yield of the desired product as a pair of isomers of 2aa ( Z/E = 19:1, Table 1 , entry 1) and a simple column chromatography separation could give the pure Z -isomer. Both the yield and stereoselectivity were reduced when the reaction was carried out in the absence of citric acid (Table 1 , entry 2). The stereoselectivity decreased to 12:1 without DPPE (Table 1 , entry 3). When the reaction was performed in the absence of KI, no desired product was obtained, which indicated that KI played a key role in this selective electro-oxidative reaction (Table 1 , entry 4). Replacing citric acid with acetic acid led to a lower yield at 79% (Table 1 , entry 5). No desired product was detected when t- BuOK was added instead of citric acid (Table 1 , entry 6). When the temperature decreased to 10 °C, a 67% yield of 2aa was found (Table 1 , entry 7). Heating the reaction mixture to 50 °C or 70 °C resulted in poor stereoselectivities (Table 1 , entries 8 and 9). Inferior reaction yield and stereoselectivity were obtained when N , N -dimethylformamide (DMF) was used as a co-solvent (Table 1 , entry 10). The influence of the electrodes was also studied. Replacing either the Pt minigrid anode or the Pt wire cathode by a Pt foil led to a poor result (Table 1 , entries 11 and 12). The increase of the electric current caused a lower yield and stereoselectivity (Table 1 , entry 13). No desired product could be detected when the reaction was carried out at a current lower than 5 mA (Table 1 , entry 14). Screening of acids or bases, redox catalysts, ligands, electrolytes, and electrode materials were also studied (See Supplementary Tables 1 – 5 ). Table 1 Optimization of reaction conditions a Full size table Substrate scope With the optimized conditions defined (Table 1 , entry 1), the scope of phenylthiols/thiols was probed. As shown in Fig. 2 , the reactions of various phenylthiols/thiols proceeded smoothly and the desired products were obtained in good to excellent yields with good stereoselectivities in most cases. First, the reactivity of phenylthiols with substituents on the benzene ring was studied. In general, both electron-donating and electron-withdrawing groups with different substitution patterns ( para- , meta- , and ortho- substitutions; mono and multi substitutions) were tolerated in this reaction. Aryl thiols bearing fluoro, chloro, bromo, methyl, and methoxy groups could give the desired products in excellent yields (90–96%) and good selectivities. In addition, other fluorine-containing phenylthiols, such as trifluoromethyl phenylthiol and pentafluoro phenylthiol, were compatible with this protocol, affording 2ad and 2f in 78 and 79% yields, respectively. Somewhat steric effects were observed with the functional groups on the ortho -position ( 2bb – 2be ). Interestingly, oxidatively labile functional groups, such as amino and hydroxy, were tolerated in this transformation to produce the corresponding products ( 2ae and 2c ) in 24 and 47% yields, respectively. The present method could also be applied to diphenyl disulfide ( 2g ). Fig. 2 Substrate scope of thiols. a Standard conditions: 1 (0.5 mmol), citric acid (10 mol%), 1,2-bis(diphenylphosphino)ethane (DPPE) (20 mol%), KI (50 mol%), MeCN (5 mL), with 0.1 M n -Bu 4 NClO 4 as electrolyte. A Pt minigrid electrode as an anode and a Pt wire as a cathode, an undivided cell, constant current = 10 mA, 4 h, room temperature. Isolated yields are shown. Z/E ratios were determined by fluorine-19 nuclear magnetic resonance ( 19 F NMR) or proton nuclear magnetic resonance ( 1 H NMR analysis). b KI (60 mol%), reaction time: 6 h. c Phenyl disulfide as a substrate. d KI (60 mol%), reaction time: 10 h. e Diselenides as substrates Full size image Naphthyl and heteroaromatic thiols ( 2 h , 2i – 2k ) were effective for this reaction. Notably, the substrate scope could also be extended to alkyl mercaptans. The primary thiols, 2-phenylethanethiol and 1-hexanethiol, could be transformed to the corresponding products ( 2 l and 2 m ) in 53 and 24% yields, respectively. The secondary thiol, that is, cyclohexanethiol gave the product ( 2n ) in a yield of 5% only. Unfortunately, no 2o was detected when benzyl mercaptan was used as the reactant. Finally, it was delightful to find that diphenyl diselenide ( 2p ) and dimethyldiselenide ( 2q ) could be converted effectively to the corresponding products in excellent yields and good selectivitities. The absolute stereochemistry of one of the products ( Z )-2ba was determined by X-ray crystallographic analysis (Fig. 2 ). The stereochemistry of other products was determined on the basis of the similarities of the polarities and the 1 H NMR and 13 C NMR chemical shifts. Next, the synthetic utility of this methodology was further investigated. First, the gram-scale synthesis of 2aa , 2ah , and 2bb was performed and the desired products were obtained in the yields of 78%, 81%, and 65%, respectively. Second, 4 H -1,4-benzothiazine scaffolds were obtained by copper-catalyzed cyclization of 2bb and the corresponding derivatives ( 3a and 3b ) in the conversion yields of 70–87%. Notably, 4 H -1,4-benzothiazine scaffolds are widely used in pharmaceutical chemistry due to their activities of antimicrobial, anticancer, and so on (Fig. 3 ). Fig. 3 Gram-scale synthesis and product transformations. Reaction conditions: (i) acetyl chloride, Et 3 N, CH 2 Cl 2 , 0 °C to reflux, 12 h, 85%; BnBr, NaH, dry N , N -dimethylformamide (DMF), N 2 , 0 °C to r.t., 4 h, 79%. (ii) CuI, K 2 CO 3 , trans - N,N′ -dimethylcyclohexane-1,2-diamine, N,N′ -dimethylethylenediamine, toluene, N 2 , 120 °C, 15 h, conditions to be optimized. a Conversions: 3c , 60%; 3d , 72%; 3e , 62% Full size image Further studies were carried out to gain more insights into the reaction mechanism. First, when a radical scavenger, TEMPO (tetramethylpiperidine N-oxyl) or BHT (butylated hydroxytoluene), was added into the reaction mixture under the standard conditions, only a trace of desired product 2aa was detected (Fig. 4a ), and thus a radical nature of the transformation was implied. On the other hand, 3-aminocrotononitrile 4 was detected by gas chromatography–mass spectrometry (GC−MS) analysis during the above two reaction processes. Subsequent investigation demonstrated that the reaction started from 4 could produce the desired product 2aa (Fig. 4b ), while no 2ab was obtained from (4-chlorophenylthio)acetonitrile 5 (Fig. 4c ). Therefore, it was confirmed that the first step of this tandem reaction is an acetonitrile self-condensation to produce 4 . Fig. 4 Mechanistic studies on the reaction. a Reactions by adding radical scavengers (tetramethylpiperidine N-oxyl (TEMPO) or butylated hydroxytoluene (BHT)). b The reaction between 1aa and 4 . c The reaction between 5 and acetonitrile Full size image Next, the formation of 4 was investigated. The pH value was monitored and it showed that the pH value increased steadily from 2 to 6 (see Supplementary Figure 1 ). Obviously, it was not a traditional Thorpe-type self-condensation through the − CH 2 CN, which usually occurs under strongly basic conditions [48] , [49] , [50] . On the other hand, a radical trapping adduct, 6 , was detected (GC−MS analysis) by the use of 1,1-diphenylethene as the radical inhibitor, which suggested the intermediacy of cyanomethyl radical (Fig. 5a ). Notably, the reaction did not proceed to afford the desired product 2aa when acetonitrile was replaced by iodoacetonitrile (Fig. 5b ). Moreover, using iodoacetonitrile instead of KI could not generate the desired product 2aa even if acetonitrile was used as a solvent (Fig. 5b ). These results rule out the formation of the intermediate ICH 2 CN in the early stage of the reaction. Fig. 5 Studies on the pathway for the formation of intermediate 4 . a Radical trapping experiment by 1,1-diphenylethylene. b The reaction between 1aa and iodoacetonitrile Full size image No desired reaction occurred in the absence of KI under the standard conditions (Table 1 , entry 4). Further studies showed that in the absence of thiol, 4 could be obtained (Fig. 6a ), while no 4 was detected without the addition of KI into the above reaction mixture. It demonstrated that KI played a crucial role in the formation of 4 . It was observed that the production of 4 needed the galvanic current, but the standard reaction could proceed in the dark (Fig. 6b ). Hence, the formation of 4 might have been catalyzed by an iodine species that was generated by anodic oxidation, instead of photoexcitation, from KI [51] , [52] . Next, to explore the actual iodine species in the reaction, several different stoichiometric amounts of iodine sources were employed in the model reaction without the current. No 4 could be detected when I 2 was applied (Fig. 6a ). It has been reported that quaternary ammonium hypoiodite [ n -Bu 4 N] + [IO] − or iodite [ n -Bu 4 N] + [IO 2 ] − could abstract a hydrogen atom from a C(sp 3 )−H to produce a radical [53] . However, the subsequent investigations using KI/TBHP, TBAI/TBHP, or I 2 /TBAOH system, which have been reported to generate hypoiodite or iodite, gave no 4 (Fig. 6a ). Thus, we hypothesized that the active iodine radical [54] , [55] , [56] , [57] , [58] , which was in situ generated from the anodic oxidation, was able to abstract one hydrogen atom from acetonitrile to form the cyanomethyl radical. Fig. 6 Studies on the active catalytic species for the formation of intermediate 4 . a I. Studies on the formation of 4 ; II. the exploration of the iodine species. 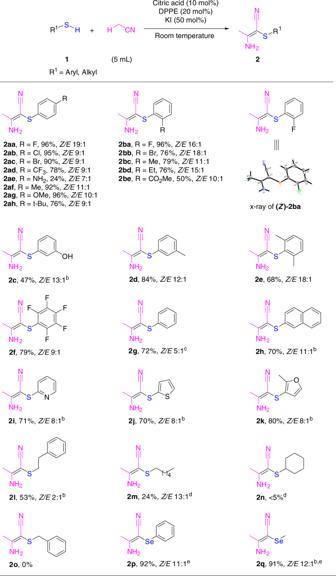Fig. 2 Substrate scope of thiols.aStandard conditions:1(0.5 mmol), citric acid (10 mol%), 1,2-bis(diphenylphosphino)ethane (DPPE) (20 mol%), KI (50 mol%), MeCN (5 mL), with 0.1 Mn-Bu4NClO4as electrolyte. A Pt minigrid electrode as an anode and a Pt wire as a cathode, an undivided cell, constant current = 10 mA, 4 h, room temperature. Isolated yields are shown.Z/Eratios were determined by fluorine-19 nuclear magnetic resonance (19F NMR) or proton nuclear magnetic resonance (1H NMR analysis).bKI (60 mol%), reaction time: 6 h.cPhenyl disulfide as a substrate.dKI (60 mol%), reaction time: 10 h.eDiselenides as substrates b The standard reaction run in dark Full size image Cyclic voltammetry studies (see Supplementary Figure 2 ) showed that KI (Fig. 7 , curve b) exhibited two pairs of typical redox waves, with the oxidation peaks at 0.46 V (Ox 1 ) and 0.80 V (Ox 2 ) vs. SCE. After acetonitrile was introduced, obvious catalytic currents were detected; the peak currents of Ox 1 and Ox 2 dramatically increased from 84 to 134 and 92 to 168 μA, respectively (Fig. 7 , curve c). Therefore, it was suggested that KI was employed as a redox catalyst in this indirect electrolysis process. Fig. 7 Cyclic voltammograms of 0.1 M n -Bu 4 NClO 4 solution in N , N -dimethylformamide (DMF) at room temperature. a None; b KI (50 mmol L −1 ); c KI (50 mmol L −1 ) + MeCN (1 mL). The voltammogram was obtained with Pt wire as an auxiliary electrode and a saturated calomel electrode (SCE) as a reference electrode. The scan rate was 0.1 V s −1 on a platinum disk electrode ( d = 2 mm) Full size image On the basis of these above results, a plausible mechanism was proposed (Fig. 8 ). The reaction sequence began with the in situ generation of an iodine radical on the anode and the iodine radical abstracted one hydrogen atom from acetonitrile to form the cyanomethyl radical 7 . Addition of 7 to another molecule of acetonitrile furnished intermediate 8 [59] . The α-imine radical intermediate 10 was obtained by a 1,3-hydrogen transfer [60] , [61] , [62] , [63] of iminyl radical 8 . Meanwhile, thiol 1aa could be oxidized by the redox catalyst or by the anode directly to afford a sulfur radical 12 , which underwent dimerization to generate a disulfide 13 [64] , [65] , [66] . Thus, radical intermediate 10 could substitute with the disulfide 13 or couple with the sulfur radical 12 directly to produce imine 11 , which could tautomerize to give the desired product 2aa in the presence of the acid catalyst. However, another pathway cannot be ruled out. Tautomerization of 10 to the corresponding enamine radical 9 was followed by the substitution with the disulfide 13 or the coupling with the sulfur radical 12 directly to form the desired product 2aa . Concomitantly, cathodic reduction of protons led to the release of H 2 . Fig. 8 Proposed mechanism. Proposed reaction mechanism involves indirect anode oxidation of acetonitrile to cyanomethyl radical 7 , addition to acetonitrile, 1,3-H transfer to produce 10 , reaction of 10 with 12 or 13 , and tautomerization to furnish the final product 2aa Full size image It was observed that the selectivity increased when DPPE was added. Studies showed that DPPE was in situ oxidized to 1,2-ethylene bis(diphenylphosphine oxide) on the anode (see Supplementary Discussion). Pre-oxidation of DPPE on the anode before the main reaction occurred the same yield and selectivity. We further carried out a density functional theory (DFT) calculations to provide insights into the mechanism (Fig. 9 ). DFT results indicate that imine type radical intermediates ( 10 or 10′ ) are more stable than the enamine type radicals ( 9 or 9′ ). The imine radical would interact with DPPE oxide to form complexes C3 – C5 , among which C3 is the most stable one with the calculated formation energies of –1.9 kcal mol −1 . The complex C3 can stabilize the yielded radical and facilitate the C–S bond formation in Z configuration. It should be noted that the enamine type products ( 2aa ) are more stable than imine types ( 11 and 11′ ). Therefore, the formed imine products would tautomerize to give the desired product 2aa , in which the ( Z )-2aa is more stable than the ( E )-2aa by 1.9 kcal mol −1 . The predicted Z : E is around 25:1, which is in excellent agreement with our experimental observation (19:1). Considering the relative stability between ( Z )-2aa and ( E )-2aa , the reaction should be thermodynamic control. DFT results suggest the important role of DPPE oxide in stabilizing the imine radical 10 , facilitating the formation of Z product and its tautomerization to final product ( Z )-2aa . Fig. 9 Density functional theory (DFT) study of the key intermediates and the calculated structures (Å, red) for complex C3 . DFT study shows imine radical 10 can be coordinated with 1,2-bis(diphenylphosphino)ethane (DPPE) oxide to form complex C3 via hydrogen bonding. The result suggests the important role of DPPE oxide in stabilizing the imine radical 10 , facilitating the formation of Z product and its tautomerization to final product ( Z )-2aa Full size image In conclusion, we have developed a radical-initiated C(sp 3 )–H bond oxidative functionalization of acetonitrile through a KI-mediated indirect anodic oxidation. A wide range of aromatic/aliphatic mercaptans bearing various functional groups could participate in the reactions with acetonitrile to afford sulfur-containing β-enaminonitrile derivatives with concomitant generation of ( Z )-tetrasustituated olefins. The high chemoselectivities and good stereoselectivities of the reactions could be achieved under metal-free, external chemical oxidant-free conditions. Further investigations into the mechanistic details and synthetic applications are currently underway in our laboratory. Representative procedure for the synthesis of 2aa Into a round bottom flask was added thiol 1aa (0.5 mmol, 1.0 equiv), KI (50 mol%), citric acid (10 mol%), and DPPE (20 mol%). MeCN (5 mL) with n -Bu 4 NClO 4 (0.1 M) as an electrolyte was then added. The resulting solution was electrolyzed with a Pt minigrid electrode (52 mesh, 1 × 1.5 cm 2 ) as anode and a Pt wire (diameter = 0.5 mm, height = 2.0 cm) as cathode, under a constant current (10 mA) in an undivided cell at room temperature for 4 h. After electrolysis, the mixture was quenched by water and extracted with ethyl acetate (3 × 10 mL). The combined organic layer was washed with brine (10 mL) and dried over Na 2 SO 4 . The ratio of ( Z ) - 2aa and ( E ) - 2aa was determined by 19 F NMR ( Z/E ratio = 19:1) of the crude mixture. 19 F NMR (377 MHz, CDCl 3 ) δ −115.97 (major), −116.73 (minor). The mixture of ( Z ) - 2aa and ( E ) - 2aa was obtained by a column chromatography separation of the crude mixture on silica gel (petroleum ether/ethyl acetate = 2:1), colorless oil, 100.0 mg, 96%. And, a further column chromatography separation could give the pure Z -isomer. Procedure for the scale-up synthesis of 2aa Into a round bottom flask was added KI (50 mol%), citric acid (10 mol%), and DPPE (20 mol%). MeCN (60 mL) with n -Bu 4 NClO 4 (0.1 M) as an electrolyte was added. Thiol 1aa (6 mmol, 1.0 equiv) was then introduced. 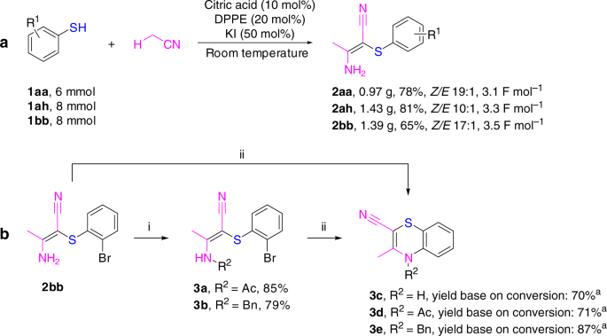Fig. 3 Gram-scale synthesis and product transformations. Reaction conditions: (i) acetyl chloride, Et3N, CH2Cl2, 0 °C to reflux, 12 h, 85%; BnBr, NaH, dryN,N-dimethylformamide (DMF), N2, 0 °C to r.t., 4 h, 79%. (ii) CuI, K2CO3,trans-N,N′-dimethylcyclohexane-1,2-diamine,N,N′-dimethylethylenediamine, toluene, N2, 120 °C, 15 h, conditions to be optimized.aConversions:3c, 60%;3d, 72%;3e, 62% The resulting solution was electrolyzed with a Pt minigrid electrode (52 mesh, 1 × 1.5 cm 2 ) as anode and a Pt wire (diameter = 0.5 mm, height = 2.0 cm) as cathode, under a constant current (10 mA) in an undivided cell at room temperature. After 50 h, the mixture was quenched by water and extracted with ethyl acetate (3 × 30 mL). The combined organic layer was washed with brine (20 mL) and dried over Na 2 SO 4 , filtered, and concentrated in vacuo. 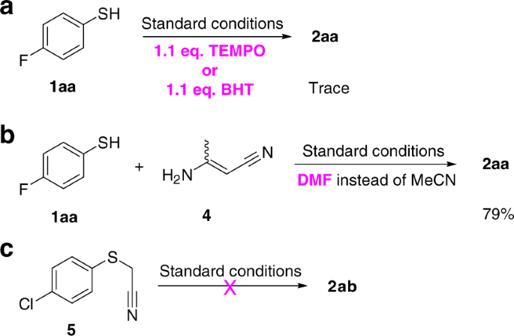Fig. 4 Mechanistic studies on the reaction.aReactions by adding radical scavengers (tetramethylpiperidine N-oxyl (TEMPO) or butylated hydroxytoluene (BHT)).bThe reaction between1aaand4.cThe reaction between5and acetonitrile 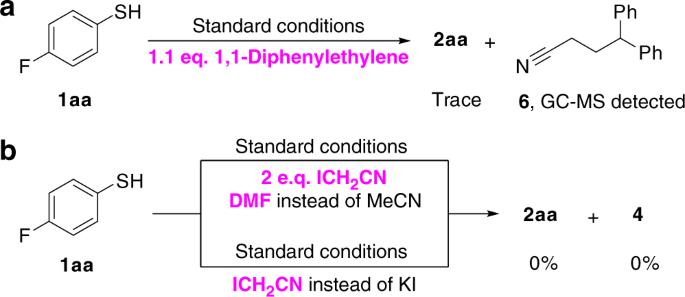Fig. 5 Studies on the pathway for the formation of intermediate4.aRadical trapping experiment by 1,1-diphenylethylene.bThe reaction between1aaand iodoacetonitrile 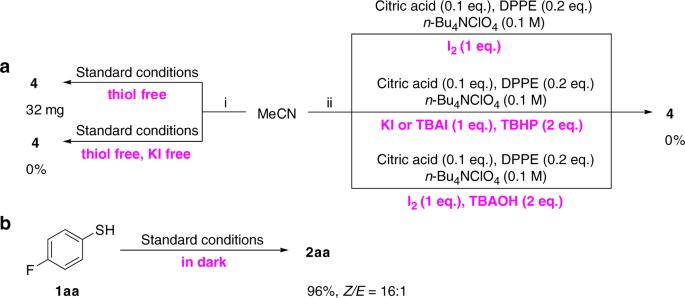Fig. 6 Studies on the active catalytic species for the formation of intermediate4.aI. Studies on the formation of4; II. the exploration of the iodine species.bThe standard reaction run in dark 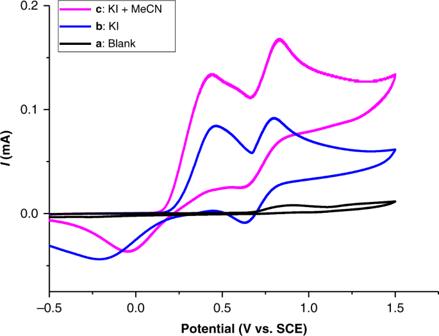Fig. 7 Cyclic voltammograms of 0.1 Mn-Bu4NClO4solution inN,N-dimethylformamide (DMF) at room temperature.aNone;bKI (50 mmol L−1);cKI (50 mmol L−1) + MeCN (1 mL). The voltammogram was obtained with Pt wire as an auxiliary electrode and a saturated calomel electrode (SCE) as a reference electrode. The scan rate was 0.1 V s−1on a platinum disk electrode (d= 2 mm) 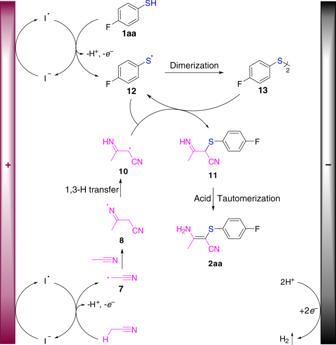Fig. 8 Proposed mechanism. Proposed reaction mechanism involves indirect anode oxidation of acetonitrile to cyanomethyl radical7, addition to acetonitrile, 1,3-H transfer to produce10, reaction of10with12or13, and tautomerization to furnish the final product2aa 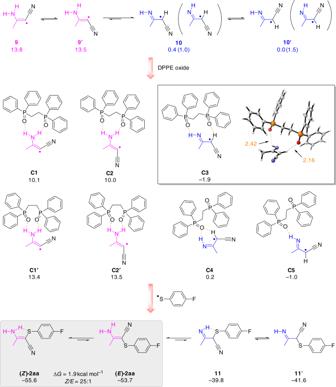Fig. 9 Density functional theory (DFT) study of the key intermediates and the calculated structures (Å, red) for complexC3. DFT study shows imine radical10can be coordinated with 1,2-bis(diphenylphosphino)ethane (DPPE) oxide to form complexC3via hydrogen bonding. The result suggests the important role of DPPE oxide in stabilizing the imine radical10, facilitating the formation ofZproduct and its tautomerization to final product(Z)-2aa The mixture of ( Z ) - 2aa and ( E ) - 2aa was obtained by a column chromatography separation of the crude mixture on silica gel (petroleum ether/ethyl acetate = 2:1), colorless oil, 0.97 g, 78%, Z/E ratio = 19:1.